Mass spectrometric analysis of mono- and multi-phosphopeptides by selective binding with NiZnFe2O4magnetic nanoparticles Selective isolation of mono- and multi-phosphorylated peptides is important for understanding how a graded protein kinase or phosphatase signal can precisely modulate the on and off states of signal transduction pathways. Here we report that metal ions at exposed octahedral sites of nano-ferrites, including Fe 3 O 4 , NiFe 2 O 4 , ZnFe 2 O 4 and NiZnFe 2 O 4 , have distinctly selective coordination abilities with mono- and multi- phosphopeptides. Due to their intrinsic magnetic properties and high surface area to volume ratios, these nanoparticles enable the rapid isolation of mono- and multi-phosphopeptides by an external magnetic field. Model phosphoprotein α-casein and two synthesized mono- and di-phosphopeptides have been chosen for proof-of-principle demonstrations, and these nanoparticles have also been applied to phosphoproteome profiling of zebrafish eggs. It is shown that NiZnFe 2 O 4 is highly selective for multi-phosphopeptides. In contrast, Fe 3 O 4 , NiFe 2 O 4 and ZnFe 2 O 4 can bind with both mono- and multi-phosphopeptides with relatively stronger affinity towards mono-phosphopeptides. Reversible protein phosphorylation is an important regulatory mechanism for prokaryotic and eukaryotic cells [1] , [2] . Cycles of phosphorylation and dephosphorylation cause conformational changes in structures of many enzymes and receptors and also function as electrostatic switches to modulate the on and off states of many signalling pathways [3] , [4] , [5] . Processive multisite phosphorylation cascades have been implicated in the regulation of many cell behaviours such as graded activity-dependent regulation of ion channel gating [6] , proper tuning of cell cycles [7] and graded enhancement of protein interactions [8] , [9] . Differentiation of mono- and multi-phosphopeptides offers compelling biological insights into their distinct functions. For example, mono- and di-phosphorylation of myosin light chain differentially regulate adhesion and polarity in migrating cells [10] ; but mono- and multisite phosphorylation of Bcl2 either enhances its antiapoptotic function or inactivates Bcl2 [11] . These experimental results suggest the functional and regulatory advantages of different levels of phosphorylation in the processing of complex cellular information. The regulated sequential or simultaneous binding of phosphate groups in multisites or just a single site with proteins may function as dynamic structural ‘codes’ in response to different physiological status or environmental stresses [12] . However, the distributions of these phospho-isoforms and the mechanisms how the dynamic structural ‘codes’ are regulated remain largely unknown. It is urgently necessary to explore new avenues that can not only isolate phosphorylated peptides from non-phosphorylated peptides, but also can further dissect the levels of phosphorylation with high resolution [13] , [14] . Magnetic nanoparticles of ferrites (mNOF) and transition metal ion doped ferrites (for example, Ni 2+ and Zn 2+ ) [15] , [16] , [17] have been studied because of their distinct magnetic and electrical properties [18] , [19] , [20] , chemical and thermal stabilities [21] , [22] , coordination abilities of exposed octahedral metal ions [22] as well as high ratios of surface area to volume. We demonstrate here that different metal ions at the surface octahedral sites of NiZnFe 2 O 4 , Fe 3 O 4 , NiFe 2 O 4 and ZnFe 2 O 4 nanoparticles have distinctly different binding affinities towards multi- and monophosphopeptides. All these features makes mNOF an ideal new tool for in-depth studies of phosphoproteomes. Selective binding of ferrites with phosphopeptides Binding of Fe 3+ or other transition metal ions with negatively charged phosphate groups has been demonstrated in IMAC (immobilized metal ion affinity chromatography) experiments [23] , [24] , [25] in which metal ions are chelated to a resin. Essentially, these metal ions can bind with both mono- and multi-phosphorylated peptides, while multi-phosphorylated peptides appear to have stronger binding affinities because of stronger electrostatic interactions. Binding affinities of metal ions present in Fe 3 O 4 , NiFe 2 O 4 , ZnFe 2 O 4 and NiZnFe 2 O 4 nanoparticles have been investigated in this work. MALDI-MS (matrix assisted laser desorption ionization-mass spectrometry) was used for methodology demonstration because it minimizes losses of multi-phosphorylated peptides that are often confronted with liquid chromatography-mass spectrometry approaches [26] . Tryptic peptides of α-casein were loaded in 50% ACN (acetonitrile) containing 0.1% TFA (trifluoroacetic acid) and eluted with 1 M ammonium phosphate as described in Methods. In contrast with IMAC, dominant peptides eluted from Fe 3 O 4 are monophosphopeptides ( Fig. 1a ), while weak peaks at m/z =2,720 and m/z =1,927 that are identified as multiphosphopeptides with either 5 or 2 phosphate groups are also detected. Similar results were observed for NiFe 2 O 4 ( Supplementary Fig. S1a ) and ZnFe 2 O 4 nanoparticles ( Supplementary Fig. S1b ). However, completely different multiphosphopeptides were found to elute from NiZnFe 2 O 4 nanoparticles ( Fig. 1b ), indicating that NiZnFe 2 O 4 has highly selective binding affinity towards multi-phosphorylated peptides. 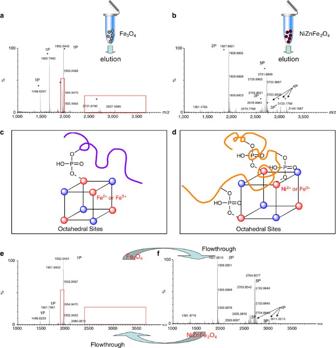Figure 1: Selective binding of Fe3O4and NiZnFe2O4nanoparticles towards mono- and multi- phosphorylated peptides. (a,b) Mass spectra of peptides directly enriched from tryptic digests of α-casein with Fe3O4and NiZnFe2O4nanoparticles. Monophosphopeptides and multi-phosphopeptides are shown as black balls and stars, respectively. Phosphorylations were labelled as P. Red squares indicate that multi-phosphorylated peptides can also be detected in the elutant from Fe3O4nanoparticles. (c,d) Binding schematic for Fe3O4and NiZnFe2O4nanoparticles. Blue balls represent oxygen atoms at cubic lattices. Metal ions at surface octahedral sites are shown as red balls. Exposed surface octahedral metal ions can provide free coordination sites to accept electron pairs donated by negatively charged phosphate groups. (e) Mass spectrum of peptides inversely enriched with Fe3O4from the flowthrough fraction of NiZnFe2O4. Red squares indicate that multi-phosphorylated peptides can not be detected after efficient NiZnFe2O4capture. (f) Mass spectrum of peptides inversely enriched with NiZnFe2O4from the flowthrough fraction of Fe3O4. Mono- phosphorylated peptides were not detected. Some unlabelled peaks with low intensities may result from in source fragmentation, formation of adducts, non-specific interactions, unknown impurities as well as interferences of peptides with carboxyl groups. False identification can be avoided by further MS/MS experiments and MASCOT database searching. In all these experiments, tryptic peptides of α-casein were loaded with nanoparticles in optimized solutions containing 50% ACN and 0.1% TFA. Figure 1c shows the binding schemes for Fe 3 O 4 and NiZnFe 2 O 4 nanoparticles, respectively. Figure 1: Selective binding of Fe 3 O 4 and NiZnFe 2 O 4 nanoparticles towards mono- and multi- phosphorylated peptides. ( a , b ) Mass spectra of peptides directly enriched from tryptic digests of α-casein with Fe 3 O 4 and NiZnFe 2 O 4 nanoparticles. Monophosphopeptides and multi-phosphopeptides are shown as black balls and stars, respectively. Phosphorylations were labelled as P. Red squares indicate that multi-phosphorylated peptides can also be detected in the elutant from Fe 3 O 4 nanoparticles. ( c , d ) Binding schematic for Fe 3 O 4 and NiZnFe 2 O 4 nanoparticles. Blue balls represent oxygen atoms at cubic lattices. Metal ions at surface octahedral sites are shown as red balls. Exposed surface octahedral metal ions can provide free coordination sites to accept electron pairs donated by negatively charged phosphate groups. ( e ) Mass spectrum of peptides inversely enriched with Fe 3 O 4 from the flowthrough fraction of NiZnFe 2 O 4 . Red squares indicate that multi-phosphorylated peptides can not be detected after efficient NiZnFe 2 O 4 capture. ( f ) Mass spectrum of peptides inversely enriched with NiZnFe 2 O 4 from the flowthrough fraction of Fe 3 O 4 . Mono- phosphorylated peptides were not detected. Some unlabelled peaks with low intensities may result from in source fragmentation, formation of adducts, non-specific interactions, unknown impurities as well as interferences of peptides with carboxyl groups. False identification can be avoided by further MS/MS experiments and MASCOT database searching. In all these experiments, tryptic peptides of α-casein were loaded with nanoparticles in optimized solutions containing 50% ACN and 0.1% TFA. Full size image In order to further confirm binding selectivities of different ferrites, flowthrough fractions of different ferrites have been inversely enriched by each other. As expected, mono-phosphorylated peptides were detected in the flowthrough fraction of NiZnFe 2 O 4 ( Fig. 1e ) and multi-phosphorylated peptides were detected in the flowthrough fraction of Fe 3 O 4 ( Fig. 1f ). Multi-phosphorylated peptides present in Fig. 1a (peaks at m/z =2,720 and m/z =1,927) were not observed in the flowthrough fraction of NiZnFe 2 O 4 ( Fig. 1e ). These experimental results demonstrate that NiZnFe 2 O 4 can selectively capture multi-phosphorylated peptides but Fe 3 O 4 can bind with both mono- and multi- phosphopeptides with relatively stronger affinities towards monophosphopeptide. Therefore, a sequential loading of samples with NiZnFe 2 O 4 followed by Fe 3 O 4 was performed in order to differentiate multi- and mono- phosphorylated peptides. By using this approach, all phosphorylation sites of α-casein was recovered ( Supplementary Table S1 ). Further separation of multi-phosphopeptides bound with NiZnFe 2 O 4 can not be achieved through gradient elution by using 20 mM, 50 mM, 100 mM and 1 M (NH 4 ) 3 PO 4 ( Fig. 2a–d ). The strong tolerance of NiZnFe 2 O 4 and Fe 3 O 4 to co-existed chemical reagents and other non-phosphorylated peptides in samples was shown in Supplementary Note 1 and Supplementary Fig. S2 . 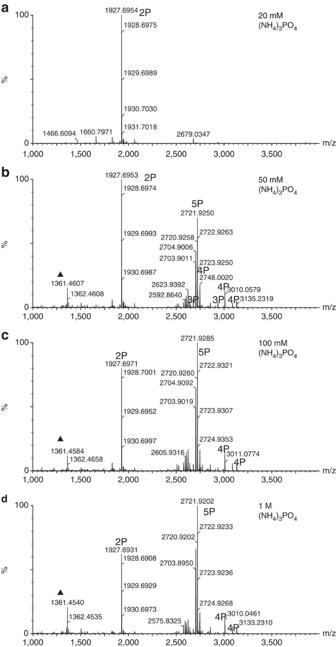Figure 2: Differences in binding affinities of NiZnFe2O4nanoparticles towards peptides with different levels of phosphorylation. (a–d) Mass spectra of multi-phosphopeptides of α-casein sequentially eluted from NiZnFe2O4nanoparticles by using gradient 20 mM (a), 50 mM (b), 100 mM (c) and 1 M (d) (NH4)3PO4, respectively. Only di-phosphopeptides atm/z=1927 is partially separated from other multi-phosphopeptides (a). Phosphopeptides with more than two phosphate groups can not be differentiated with NiZnFe2O4nanoparticles. Black triangles represent interferences of unknown peaks. Figure 2: Differences in binding affinities of NiZnFe 2 O 4 nanoparticles towards peptides with different levels of phosphorylation. ( a – d ) Mass spectra of multi-phosphopeptides of α-casein sequentially eluted from NiZnFe 2 O 4 nanoparticles by using gradient 20 mM ( a ), 50 mM ( b ), 100 mM ( c ) and 1 M ( d ) (NH 4 ) 3 PO 4 , respectively. Only di-phosphopeptides at m/z =1927 is partially separated from other multi-phosphopeptides ( a ). Phosphopeptides with more than two phosphate groups can not be differentiated with NiZnFe 2 O 4 nanoparticles. Black triangles represent interferences of unknown peaks. Full size image Effects of experimental conditions The experimentally optimized loading condition for Fe 3 O 4 and NiZnFe 2 O 4 is a solution containing 50% ACN and 0.1% TFA ( Fig. 1 ). Both pH value and the organic solvent have critical roles in the binding specificities. As for Fe 3 O 4 , three non-phosphopeptides including HIQKEDVPSER (1,337 Da), HQGLPQEVLNENLLR (1,759 Da) and EPMIGVNQELAYFYPELFR (2,316 Da) as well as an impurity peak at m/z =1,116 Da were observed under a weaker acidic condition of 0.01% TFA ( Supplementary Fig. S3a ). All three peptides has at least two glutamic acid residues that can provide carboxyl groups to interact with metal ions. Loading of samples in solutions without acetonitrile also causes non-specific binding ( Supplementary Fig. S3b ). Delightedly, Fe 3 O 4 has strong tolerance to 0.01% SDS ( Supplementary Fig. S3c ) or even 0.1% SDS ( Supplementary Fig. S3d ) that is commonly used for biological sample preparations. The same sample loading conditions have been evaluated for NiZnFe 2 O 4 . It was shown that pH value ( Supplementary Fig. S3e ), organic solvent composition ( Supplementary Fig. S3f ) and SDS concentration ( Supplementary Fig. S3g,h ) do not significantly affect the binding selectivity of NiZnFe 2 O 4 towards multi-phosphopeptides. However, signal-to-noise ratios in Supplementary Fig. S3e–h are significantly lower than that in optimized condition ( Fig. 1 ). It means that experimental conditions do exert effects on recoveries of multi-phosphopeptides. Similar results were observed for NiFe 2 O 4 ( Supplementary Fig. S4 ) and ZnFe 2 O 4 ( Supplementary Fig. S5 ). But Fe 3 O 4 and NiZnFe 2 O 4 were chosen for downstream sample analysis because they have better magnetic properties than NiFe 2 O 4 and ZnFe 2 O 4 . Assessment of the binding performance of NiZnFe 2 O 4 The intrinsic difficulties of MALDI mass spectrometer in ion suppression, ionization and especially heterogeneous crystallization of DHB matrix (2, 5-dihydroxybenzoic acid) limit its application to quantitative analysis by using absolute intensities. In order to quantitatively assess the detection limit, two synthesized peptides P1 and P2 (in 1:1 molar ratio) with 1 or 2 phosphate groups were loaded with NiZnFe 2 O 4 nanoparticles and eluted with 1 M (NH 4 ) 3 PO 4 . After ZipTip desalting, the final elutant was mixed with CHCA (α-cyano-4-hydroxycinnamic acid) instead of DHB for MALDI analysis here. The detection limit of NiZnFe 2 O 4 can be down to 0.3 pmol with a reasonable S/N ratio, while the high selectivity towards multi-phosphopeptides is still remained ( Supplementary Fig. S6 ). It should be indicated that the detection limit is not only associated with enrichment methods but also highly related with sample preparation methods and instruments. In addition, although DHB undergoes heterogeneous crystallization, it is better than CHCA for ionization of phosphopeptides. On the basis of these considerations, higher amounts of samples and DHB are recommended for sample analysis in order to reproducibly generate high quality MS and MS/MS spectra for further database searching. The recoveries and selectivity of NiZnFe 2 O 4 towards multi-phosphopeptides were quantitatively assessed by using a LC approach based on peak areas at 214 nm. As the detection limit of LC is in the level of nmol that is much higher than that of mass spectrometry, it provides a useful means for testing the capacities of NiZnFe 2 O 4 nanoparticles to selectively isolate multi-phosphopeptides in the presence of huge amounts of monophosphopeptides. A mixture containing 3 nmol of P2 and 3 nmol of P1 was loaded with NiZnFe 2 O 4 nanoparticles. For three repeated experiments, recoveries of P2 were 87%, 88% and 85% but recoveries of P1 were only 1.4%, 1.2% and 1.5%, respectively ( Supplementary Fig. S7 ). The performance of NiZnFe 2 O 4 has also been compared with other approaches including TiO 2 [27] , [28] , [29] , [30] , Fe 3+ -IMAC [31] and HAP (hydroxyapatite) [32] , [33] ( Supplementary Note 2 ; Supplementary Table S2 ). These materials can bind with both mono- and multi- phosphorylated peptides without selectivity ( Supplementary Fig. S8 ). Partial separations of peptides with different degrees of phosphorylation can only be achieved through sequential elutions by using different solvents ( Supplementary Figs S9–S11 ). Phosphoproteome profiling of zebrafish eggs As zebrafish share significant similarities in developmental processes with human and other vertebrates, it has emerged as an ideal model to study environmental exposures and risks for developing diseases [34] . In particular, the external fertilization of zebrafish eggs offers additional benefits for such studies. Analysis of changes in protein phosphorylation should be able to reveal the cues for toxic effects of environmental pollutants on fertilization and embryo development [35] , [36] . Tryptic peptides of zebrafish egg proteins were first loaded with NiZnFe 2 O 4 and then the flowthrough fraction was loaded with Fe 3 O 4 . All enriched phosphopeptides were one-step eluted out with 1 M (NH 4 ) 3 PO 4 and two distinct peptide pools ( Fig. 3a ; Supplementary Table S3 ) were obtained. For better separation, multi-phosphopeptides bound with NiZnFe 2 O 4 were also sequentially eluted out by using gradient 20 mM, 50 mM and 100 mM (NH 4 ) 3 PO 4 ( Supplementary Fig. S12 ). It is not surprising that dominant peaks eluted from NiZnFe 2 O 4 are multi-phosphorylated peptides ( Fig. 3a ). Several peptides from vitellogenin are found to be highly multi-phosphorylated. Vitellogenin is not only a major precursor of egg-yolk proteins crucial for successful embryonic and larval growth but also has been considered as a useful biomarker for detecting the oestrogenic activity of chemicals in acquatic environments [37] . The biological roles of different levels of phosphorylation events on this protein remain largely unknown [38] . The peak at m/z =1,964 was unambiguously identified as DT SS G S AAA S FEQMQK with four phosphate groups (Phosphorylated amino acids were indicated by bold characters). A series of peaks with losses of 80 Da masses including m/z =1,884, m/z =1,804 and m/z =1,724 support the presence of multiple phosphate groups. These peaks may result from in source fragmentation that is usually observed in mass spectrometric analysis. An interesting example is the peak at m/z =2,749 that was identified as THHGD S K SS R ST G S SLEQIQK with five phosphate groups on all serines except the last one [39] . Although the peak at m/z =2,829 was not successfully identified, the 80 Da mass difference indicates that the last S in this peptide was also phosphorylated. Some other peaks were also not successfully identified due to low abundance or inefficient fragmentation. However, the presence of peaks with losses of 80 Da masses suggests that these peptides have undergone extensive multiphosphorylation. Two obvious series of such peptides include the peaks at m/z =3,928, 3,848, 3,768, 3,688, 3,608, 3,528 and the peaks at m/z =3,905, 3,825, 3,745 and 3,665. Although losses of 80 Da masses are helpful to locate multi-phosphopeptides, the identification of monophosphopeptides becomes challenging. There are no experimental evidences to confirm if monophosphopeptides are produced in source or in vivo. In Fig. 3a , the peak at m/z =1,724 is identified as a monophosphopeptide DTSSG S AAASFEQMQK. However, the formation of this monophosphopeptide is unknown [39] . Fortunately, the flowthrough fraction of NiZnFe 2 O 4 has been subsequently enriched with Fe 3 O 4 ( Fig. 3b ). The peak at m/z =1,724 becomes the dominant peak which confirms the in vivo production. Other peptides eluted from Fe 3 O 4 such as peaks at m/z =3,276, 3,526, 3,955 and 3,417 have also been unambiguously identified as monophosphopeptides. Without enrichment by NiZnFe 2 O 4 or Fe 3 O 4 , none of these phosphorylated peptides can be observed ( Supplementary Fig. S13 ). 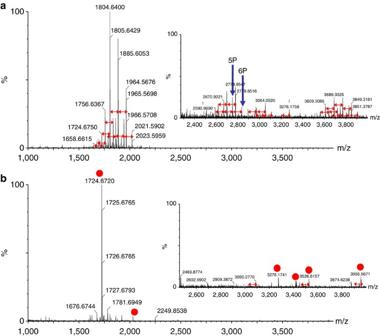Figure 3: Phosphoproteome profiling of zebrafish eggs. (a) Mass spectrum of multi-phosphorylated peptides enriched with NiZnFe2O4nanoparticles directly from the tryptic digests of zebrafish egg proteins. The blue arrows indicates the peptides containing five and six phosphate groups. (b) Mass spectrum of mono-phosphorylated peptides (labelled as red balls) enriched with Fe3O4from the flowthrough fraction of NiZnFe2O4nanoparticles. Losses of 80 Da masses were observed probably owing to in source fragmentation, especially for multi-phosphorylated peptides (labelled as red arrows). Figure 3: Phosphoproteome profiling of zebrafish eggs. ( a ) Mass spectrum of multi-phosphorylated peptides enriched with NiZnFe 2 O 4 nanoparticles directly from the tryptic digests of zebrafish egg proteins. The blue arrows indicates the peptides containing five and six phosphate groups. ( b ) Mass spectrum of mono-phosphorylated peptides (labelled as red balls) enriched with Fe 3 O 4 from the flowthrough fraction of NiZnFe 2 O 4 nanoparticles. Losses of 80 Da masses were observed probably owing to in source fragmentation, especially for multi-phosphorylated peptides (labelled as red arrows). Full size image The same samples have been analysed by Fe 3+ -IMAC ( Supplementary Fig. S14 ), HAP ( Supplementary Fig. S15 ) and TiO 2 approaches [39] . Different degrees of co-elution of mono- and multi- phosphopeptides were observed. Mechanisms of these methods are different and they are all useful tools for exploration of complex biological samples with different research goals. MASCOT searching results were listed in Supplementary Figs S16–S29 . Some peptides that have been previously identified by MS/MS database searching [39] were only identified by MS experiments in the work. All experimental results show that nanostructured magnetic ferrites, including Fe 3 O 4 , NiFe 2 O 4 , ZnFe 2 O 4 and NiZnFe 2 O 4 , have distinct selectivities towards mono- and multi- phosphorylated peptides. Cubic ferrites have well established spinel structure that is based on a face centred cubic lattice of oxygen ions, forming tetrahedral and octahedral coordination sites [40] , [41] . Binding of phosphate groups is dependent on the distribution of metal ions at the surface octahedral sites [40] . Fe 3 O 4 has an inverse spinel structure in which Fe 2+ and half Fe 3+ ions are arranged in octahedral sites and another half Fe 3+ ions are arranged in tetrahedral sites [42] . Selective binding of monophosphopeptides with Fe 3 O 4 indicates that either Fe 2+ or Fe 3+ at the surface can not efficiently bind with multi-phosphopeptides. Substitution of Fe 2+ by magnetic divalent cation Ni 2+ maintains the inverse spinel structure [43] . In resultant NiFe 2 O 4 , Ni 2+ and half Fe 3+ ions occupy the octahedral sites and another half Fe 3+ ions occupy the tetrahedral sites similar as that in Fe 3 O 4 . But the replacement of surface Fe 2+ ions by Ni 2+ ions alone does not cause significant changes in the binding affinities towards phosphopeptides. Further substitution of Fe 2+ by diamagnetic divalent cation Zn 2+ results in the formation of a normal spinel structure in which Zn 2+ ions occupy the tetrahedral sites and all Fe 3+ occupy the octahedral sites [44] . However, the incorporation of Zn 2+ also can not make detectable changes. Resultant ZnFe 2 O 4 still remains similar binding affinities as that of Fe 3 O 4 and NiFe 2 O 4 . In contrast, NiZnFe 2 O 4 shows distinct binding selectivity towards multi-phosphorylated peptides. It has mixed Fe 3+ /Ni 2+ ions at the octahedral sites and mixed Fe 3+ /Zn 2+ ions at the tetrahedral sites [45] . The experimental results suggest that interactions of cations on octahedral and tetrahedral sites in spinels may contribute to the selective binding affinities towards multi-phosphopeptides [46] . It has been reported that the substitution of iron by zinc decreases the area of tetrahedral sublattice as well as the magnetic field of octahedral sublattice but increases the area of octahedral sublattice [47] . As a result, there maybe less steric effects and less instable motions caused by the magnetic field when negatively charged multi-phosphopeptides bind with cations at the surface octahedral sites. In summary, there are mainly two factors that determine the overall coverage of phosphorylation sites by using mNOF. First, the binding affinity of metal ions at surface octahedral sites with phosphopeptides depends on the interactions between negatively charged phosphate groups and positively charged metal ions. Metal ions at the surface octahedral sites offer free coordination sites to accept electron pairs provided by phosphate groups. According to the principle of hard and soft acids and bases described by Pearson [48] , Fe 3+ is classified as a hard Lewis acid. Therefore, Fe 3+ theoretically has a strong binding with phosphorylated amino acids that are classified as hard Lewis bases. In this study, all ferrites have Fe 3+ or together with Ni 2+ at the surface octahedral sites, providing the fundamental structure to coordinate with negatively charged phosphate groups. Second, the selectivity of ferrites towards mono- and multi-phosphorylated peptides is dependent on the interactions of cations at the octahedral and tetrahedral sites. NiZnFe 2 O 4 is highly selective towards multi-phosphopeptides probably because of the increased area and decreased magnetic field of exposed surface octahedral sublattices. Preparation of magnetic nanoparticles of ferrites NiZnFe 2 O 4 nanoparticles were purchased from Sigma-Aldrich. Fe 3 O 4 , NiFe 2 O 4 and ZnFe 2 O 4 nanoparticles were prepared by a chemical co-precipitation method described as follows. Otherwise all these nanoparticles can be purchased from Sigma-Aldrich. Stock solutions of 1 M FeCl 3 , FeCl 2 , ZnSO 4 and Ni (NO 3 ) 2 were prepared in 2 M HCl, respectively. Mix 10 ml of 1 M FeCl 3 solution with 5 ml of 1 M FeCl 2 solution solely, or together with either 5 ml of 1 M ZnSO 4 or Ni (NO 3 ) 2 solutions at room temperature in order to make ferrites doped with different metal ions. Add ammonium hydroxide to the mixtures drop by drop with stirring until the pH value of the solutions reached 11–12. Keep stirring at room temperature for 30 min. And then the magnetic nanoparticles were washed three times with water and subsequent three times with ethanol. The morphology of resultant nanoparticles of ferrites has been characterized by Scan Electron Microscope (JEOL, Japan). It was observable that these nanoparticles are essentially uniform. All resultant nanoparticles can be stably dispersed into the sample loading buffer and washing buffer containing 50% ACN and 0.1% TFA. Therefore, these nanoparticles are readily accessible to biological samples and can efficiently interact with electron donor groups present in samples. In particular, these nanoparticles not only provide immobilized metal ions such as, Fe 3+ and Ni 2+ as well as high ratio of surface area to volume for efficient entrapment of phosphopeptides, but they also offer intrinsic magnetic properties to enable rapid isolation of target molecules from a complex mixture within few seconds by a magnetic field. The magnetic nanoparticles were kept with ethanol in a 4 °C fridge for the following experiments. Before use, these nanoparticles should be washed with pure water. Enrichment of model phosphopeptides with ferrites Model phosphoprotein α-casein (5 μg μl −1 ) or non-phosphoprotein cytochrome c (5 μg μl −1 ) was tryptically digested in 100 mM NH 4 HCO 3 at a concentration of 50:1 (protein versus trypsin) for 12 h in a 37 °C water bath. The final concentration of tryptic peptides was 0.5 μg μl −1 . Taken 30 μl of tryptic peptides to mix with 100 μl of ACN, 69 μl of pure water and 1 μl of 20% TFA, so the final loading buffer contained 50% ACN and the pH value was about 1–2. Then 5 mg of magnetic nanoparticles of different ferrites were added to the mixture. After vortex the mixture for 60 min, the nanoparticles were collected by an external magnetic field. And then the supernatant was discarded. The nanoparticles were first washed three times with the loading buffer containg 50% ACN and 0.1% TFA. In order to elute enriched phosphopeptides, washed nanoparticles were first re-suspended in 100 μl of 1 M ammonium phosphate solution and vortexed for 3 min. After collected the supernatant, nanoparticles were then re-suspended in 50 μl of 1 M ammonium phosphate solution again and vortexed for another 3 min. Combine all the supernatants into an Eppendorf vial for following MALDI-MS/MS experiments. To obtain a better separation, phosphopeptides have also been gradiently eluted out by using sequential 20 mM, 50 mM, 100 mM and 1 M ammonium phosphate solutions, respectively. In order to evaluate the binding specificities of different ferrites with mono- and multi-phosphopeptides, the flowthrough fractions of Fe 3 O 4 and NiZnFe 2 O 4 have been inversely enriched by NiZnFe 2 O 4 and Fe 3 O 4 , respectively. All downstream procedures such as loading, washing and elution were the same as that described above. Enrichment of zebrafish egg phosphopeptides with ferrites Zebrafish eggs were washed three times with 0.675% saline solution over ice. Then 200 zebrafish eggs were lysed with 200 μl lysis buffer that was purchased from Shenergy Biocolor BioScience and Technology (Shanghai, China) in a glass tissue homogenator. The lysis buffer was used together with protease inhibitor containing PMSF (100 mM), Aprotinin (15 μM), Leupeptin (100 μM), Bestatin (100 μM), Pepstatin A (100 μM), E-64 (80 μM). The non-soluble tissue debris was removed by centrifugation at 16,000 g for half hour at 4 °C and the supernatant was pipetted into an Eppendorf vial. Protein concentration was determined by Bradford protein assay reagent according to the manufacturer’s instruction. About 1 mg proteins of zebrafish eggs were reduced by dithiothreitol, derived by iodoacetamide and tryptically digested in 0.1 M NH 4 HCO 3 solution at a concentration of 50:1 (protein versus enzyme) for 12 h in a 37 °C water bath. The final concentration of tryptic peptides is 2 μg μl −1 . Pipette 300 μg tryptic peptides into two vials containing 10 mg nanoparticles of Fe 3 O 4 and NiZnFe 2 O 4 , respectively. Add acetonitrile and TFA into the vials so that the final loading buffer contained 50% acetonitrile and 0.1% TFA. Similarly, the flowthrough fractions have also been inversely enriched by NiZnFe 2 O 4 and Fe 3 O 4 . The other procedures for sample loading, washing and elution were the same as that used for the model protein casein. Phosphopeptides have also been eluted out gradiently by using sequential 20 mM, 50 mM, 100 mM and 1 M ammonium phosphate solutions, respectively. Enrichment of phosphopeptides with TiO 2 , HAP and Fe 3+ -IMAC The same amount of tryptic peptides of casein or zebrafish egg proteins was also analysed with 5 mg TiO 2 , HAP and Fe 3+ -IMAC. TiO 2 particles were synthesized by using a sol-gel method [39] . For TiO 2 and Fe 3+ -IMAC approach, the loading buffer contains 50% acetonitrile and 0.1% TFA. For HAP approach, the loading buffer contains 20 mM Tris–HCl (pH ~7.2) and 20% acetonitrile. The loading time for all samples was 60 min. All beads were separated by centrifugation at 16,000 g for 5 min. For TiO 2 approach, the supernatant was discarded and TiO 2 particles were sequentially re-suspended in 20 mM, 50 mM, 100 mM and 1 M (NH 4 ) 3 PO 4 solutions, respectively, in order to gradiently elute out different phosphopeptides. Alternatively, phosphopeptides were one-step eluted out with 1 M (NH 4 ) 3 PO 4 solution. Then phosphopeptides were desalted with Millipore C18 ZipTip (MA, USA) and sequentially eluted out by using 5, 10, 20, 30, 50 and 80% acetonitrile solution containing 0.1% TFA. For HAP approach, the supernatant was discarded and phosphopeptides were sequentially eluted out from HAP particles with 20 mM, 50 mM, 100 mM and 1 M Na 2 HPO 4 (pH ~7.2). For Fe 3+ -IMAC approach, phosphopeptides present in the supernatant was enriched with TiO 2 and eluted out with 1 M (NH 4 ) 3 PO 4 . Phosphopeptides bound with IMAC gels were washed with 20% acetonitrile containing 1% TFA and eluted out with 0.5% ammonia water. Mass spectrometric analysis Before mass spectrometric analysis of phosphopeptides, Millipore C18 ZipTip (MA, USA) was used to desalt the elutants containing concentrated salts such as (NH 4 ) 3 PO 4 or Na 2 HPO 4 . The ZipTip was first wetted with 50% acetonitrile and equilibrated with 0.1% TFA in H 2 O. Add 20% TFA to the elutant in order to reach a pH ~2. And then acidified elutant was loaded into the ZipTip. After three cycles of wash with 0.1% TFA in H 2 O, phosphopeptides were directly eluted out with 4 μl of 1 M DHB solution containing 50% acetonitrile and 0.1% TFA. And each of 0.8 μl elutant was deposited onto the MALDI plate for full scan MS experiments and MS/MS experiments. In order to identify as many unknown proteins in zebrafish eggs as possible, each sample has been deposited into several spots so as to acquire as many MS/MS spectra as possible. The MALDI experiments were performed on a MALDI Synapt G2 HDMS system (Waters, USA) in the sensitivity mode (V mode). (Glu1)-Fibrinopeptide B was used as the lock-mass for instrumental calibration. All MS spectra and MS/MS spectra were interpreted manually according to the known sequence of the model proteins or by MASCOT searching for unknown proteins in zebrafish eggs. Quantification of the binding performance of NiZnFe 2 O 4 Two synthesized peptides were purchased from APeptide Co. Ltd (Shanghai, China) including Cys-Ser-Lys-Asn-Gln-Ile- Ser(p) -Thr-Leu-Asp-Phe-Ser (P1) and Cys-Arg-Gly-Val-His-His-Ile-Asp- Tyr(p) - Tyr(p) -Lys-Lys-Thr-Ser-Asn (P2). They were mixed together in 1:1 molar ratio. In order to prevent the formation of disulphide bonds, free thiol groups of these synthesized peptides were blocked with NEM ( N -ethylmaleimide). Then 10 mg of NiZnFe 2 O 4 nanoparticles were loaded with the mixture containing 3 nmol of P1 and 3 nmol of P2 (equivalent to 4 μg of P1 and 6 μg of P2) in a loading buffer (50% ACN and 0.1% TFA) for 1 h. And then these nanoparticles were extensively washed with the loading buffer and finally eluted out with 1 M (NH 4 ) 3 PO 4 solution. The eluted peptides or standard peptides were first acidified with 20% TFA until pH 2~3 before they were injected into an Agilent 1100 HPLC system equipped with a Kromasil C8 chromatographic column (4.6 × 150 mm, 5 μm, 300 A°) for separation. Peaks were detected at 214 nm and peak areas were obtained through an automatic integration. To determine the detection limit of NiZnFe 2 O 4 nanoparticles, the same process of sample loading, washing, elution and acidification as described above was performed. The phosphopeptides were then desalted by using a Millipore C18 ZipTip before mixed with CHCA matrix for MALDI analysis. Each sample spot contains 30, 3 and 0.3 pmol of synthesized phosphopeptides P1 and P2, respectively. How to cite this article: Zhong, H. et al . Mass spectrometric analysis of mono- and multi- phosphopeptides by selective binding with NiZnFe 2 O 4 magnetic nanoparticles. Nat. Commun. 4:1656 doi: 10.1038/ncomms2662 (2013).